A quantum circuit rule for interference effects in single-molecule electrical junctions A quantum circuit rule for combining quantum interference effects in the conductive properties of oligo(phenyleneethynylene) (OPE)-type molecules possessing three aromatic rings was investigated both experimentally and theoretically. Molecules were of the type X-Y-X, where X represents pyridyl anchors with para (p), meta (m) or ortho (o) connectivities and Y represents a phenyl ring with p and m connectivities. The conductances G XmX ( G XpX ) of molecules of the form X-m-X (X-p-X), with meta (para) connections in the central ring, were predominantly lower (higher), irrespective of the meta, para or ortho nature of the anchor groups X, demonstrating that conductance is dominated by the nature of quantum interference in the central ring Y. The single-molecule conductances were found to satisfy the quantum circuit rule G ppp / G pmp = G mpm / G mmm . This demonstrates that the contribution to the conductance from the central ring is independent of the para versus meta nature of the anchor groups. Studies of the electrical conductance of single molecules attached to metallic electrodes not only probe the fundamentals of quantum transport but also provide the knowledge needed to develop future molecular-scale devices and functioning circuits [1] , [2] , [3] , [4] , [5] , [6] , [7] , [8] , [9] . Owing to their small size (on the scale of Angstroms) and the large energy gaps (on the scale of eV), transport through single molecules can remain phase coherent even at room temperature, and constructive or destructive quantum interference (QI) can be utilized to manipulate their room temperature electrical [10] , [11] , [12] , [13] and thermoelectrical [14] , [15] properties. In previous studies, it was reported theoretically and experimentally that the conductance of a phenyl ring with meta (m) connectivity is lower than the isomer with para (p) connectivity by several orders of magnitude [16] , [17] , [18] , [19] , [20] , [21] , [22] , [23] , [24] , [25] . This arises because partial de Broglie waves traversing different paths through the ring are perfectly out of phase leading to destructive QI in the case of meta coupling, while for para or ortho coupling they are perfectly in phase and exhibit constructive QI. (See, for example, equation 8 of ref. 26 .) It is therefore natural to investigate how QI in molecules with multiple aromatic rings can be utilized in the design of more complicated networks of interference-controlled molecular units. The basic unit for studying QI in single molecules is the phenyl ring, with thiol [17] , [21] , methyl thioether [27] , amine [17] or cyanide [19] anchors directly connecting the aromatic ring to gold electrodes. Recently, Arroyo et al . [28] , [29] studied the effect of QI in a central phenyl ring by varying the coupling to various anchor groups, including two variants of thienyl anchors. However, the relative importance of QI in central rings compared with QI in anchor groups has not been studied systematically because the thienyl anchors of Arroyo et al . [28] , [29] were five-membered rings, which exhibit only constructive interference. To study the relative effect of QI in anchors, we examined molecules with terminal groups formed from six-membered pyridyl rings for which constructive and destructive interference is possible. We have previously reported that pyridyl rings are excellent anchor groups for attaching single molecules to metallic electrodes because of their well-defined binding geometry [30] , in which the nitrogen plays the role of the anchoring site. The ability to substitute pyridine either para (p), meta (m) or ortho (o) to the nitrogen offers the possibility of systematically investigating the relative importance of QI in this anchor group in molecules of the type X-Y-X, where X is a pyridyl ring and Y is a central phenyl ring. This question is rather subtle because charge transport from the electrode into the pyridyl rings takes place via the N atom and also via metal–π coupling [31] and the interplay between these two mechanisms will determine the importance and robustness of QI in the terminal [32] rings. In the present paper, our aim is to compare the effects of QI in both the terminal rings X and the central ring Y of molecules of the type X-Y-X, and to study the relationship between their conductances. Our results were found to satisfy the quantum circuit rule G ppp / G pmp = G mpm / G mmm , which demonstrates that the contribution to the conductance from the central ring is independent of the para versus meta nature of the anchor groups. Combinatorial rules for QI in molecules with other geometries including fused rings or rings connected in parallel are discussed in refs 33 , 34 , 35 , 36 . We studied the pyridyl-terminated oligo(phenyleneethynylene) (OPE) derivatives shown in Fig. 1 , which possess a variety of connectivities of the central ring and locations of the nitrogen in the anchor units. In group 1, the central unit Y is a phenyl ring with para connectivity, whereas the central ring of group 2 has meta connectivity. The anchor units X are pyridyl rings with their nitrogens located in either meta, ortho or para positions. 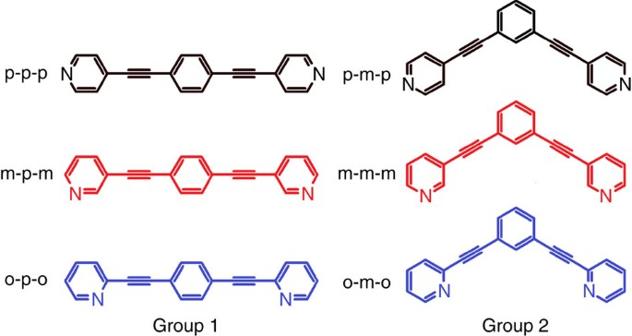Figure 1: The molecular structures studied in this paper. These are divided into two groups, based on the presence of a para (group 1) or meta (group 2) central phenyl ring. Figure 1: The molecular structures studied in this paper. These are divided into two groups, based on the presence of a para (group 1) or meta (group 2) central phenyl ring. Full size image Break-junction experiments Charge transport characteristics of single-molecule junctions formed from the molecules in Fig. 1 were investigated using both the mechanically controllable break-junction (MCBJ) and scanning tunnelling microscopy break-junction (STM-BJ) techniques, as reported elsewhere [6] , [30] , [37] , [38] . Nuclear magnetic resonance spectra for these molecules and details of synthesis are presented in Supplementary Note 1 and Supplementary Figs 1–6 . 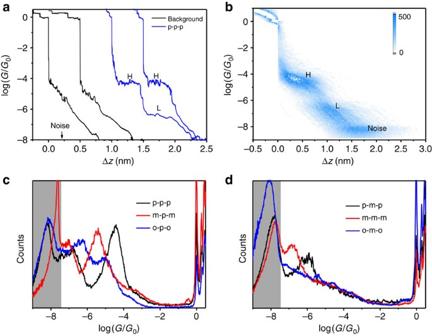Figure 2: Conductance measurements. (a) Typical individual conductance–distance traces of p-p-p (blue) and pure tunnelling traces (black). (b) All-data-point 2D conductance versus relative distance (Δz) of p-p-p. (c,d) All-data-point 1D conductance histograms constructed from 1,000 MCBJ traces of molecules in group 1 (c) and in group 2 (d). The grey area is the noise level. Figure 2a displays typical traces of the conductance G (in units of the conductance quantum G 0 =2 e 2 /h ) versus the relative electrode displacement (Δ z ) from measurement of the molecule p-p-p. Corresponding results for other molecules are presented in Supplementary Note 2 and Supplementary Figs 7–12 . Δ z is defined to be zero when G= 0.7 G 0 . It is related to the electrode separation z exp. by z exp. =Δ z +Δ z corr , where the correction Δ z corr =0.5±0.1 nm accounts for the snap-back of the electrodes upon breaking of the gold–gold atomic contact [39] . For this molecule, the log( G / G 0 ) versus Δ z stretching traces possess well-defined plateaus in the range of log( G / G 0 ) around −4.5, which we assign to the conductance of single-molecule junctions. The two-dimensional (2D) histograms of p-p-p in Fig. 2b show features of gold point contacts around G ≥1 G 0 followed by a second accumulation in the cloud-like scatter plot in the range (10 −5.0 G 0 < G <10 −3.6 G 0 ), centred at G =10 −4.5 G 0 . We attribute the latter to the formation of single-molecule junctions. These clouds of conductance data lead to peaks in the corresponding one-dimensional (1D) conductance histogram. The cloud-like pattern is observed in both MCBJ and STM-BJ measurements and the 1D histogram peaks are in good agreement with each other. Figure 2c,d displays the corresponding 1D conductance histograms of molecules belonging to groups 1 and 2 in a semi-logarithmic scale, constructed from 1,000 experimental conductance–distance traces for each compound. Figure 2: Conductance measurements. ( a ) Typical individual conductance–distance traces of p-p-p (blue) and pure tunnelling traces (black). ( b ) All-data-point 2D conductance versus relative distance (Δ z ) of p-p-p. ( c , d ) All-data-point 1D conductance histograms constructed from 1,000 MCBJ traces of molecules in group 1 ( c ) and in group 2 ( d ). The grey area is the noise level. Full size image The sharp peaks ~1 G 0 represent the conductance of a single-atom gold–gold contact. The prominent peaks between 10 −7 G 0 < G <10 −4 G 0 represent molecular conductance features. Significant difference of single-molecule conductances are observed from the variety of connectivities of the central ring ( Fig. 2c ) and locations of the nitrogen in the anchor units ( Fig. 2d ), while para connection in both central and terminal rings shows the highest conductance in both cases. The statistically most-probable conductance values were obtained by fitting Gaussians to the maxima in the conductance histograms. Our key results are summarized in Table 1 . In anticipation of the theoretical discussion below, it is interesting to note that to within experimental error, log( G ppp / G 0 )+log( G mmm / G 0 ; that is, −4.5 to 6.9) is equal to log( G pmp / G 0 )+log( G mpm / G 0 ; that is, −5.5 to 6.0), which suggests that the product of the conductances for p-p-p and m-m-m molecules is equal to the product of conductances for p-m-p and m-p-m molecules, and the quantum circuit rule G ppp / G pmp = G mpm / G mmm is satisfied. Table 1 Most-probable experimental conductance, electrode separation z H * at the end of the high-conductance plateaus and JFP of pyridyl-terminated OPE derivatives from MCBJ and STM-BJ. Full size table Further statistical analysis of conductance versus Δ z curves provides information about the junction formation probability (JFP) and allows us to determine the most-probable relative electrode displacement (Δ z H *) at the end of the high-conductance plateaus. For every log (G/G 0 ) versus Δ z stretching trace, we determine the relative electrode displacement at the end of the high-conductance plateau, Δ z H , which is the largest Δ z value within the range −0.3>log( G / G 0 )>log( G H end / G 0 ), where G H end is the end of high-conductance feature. The most-probable values of Δ z H (denoted Δ z H *) are obtained by constructing a histogram and fitting a Gaussian function to the largest maxima. Taking into account the snap-back length, the most-probable electrode separations at the end of the high-conductance plateau are z H *=Δ z H *+ Δz corr . The representative Δ z H histograms with Gaussian fitting functions are shown in Supplementary Figs 7–12 . The JFP is calculated as the ratio of the area under the fitted Gaussian function and the total area of the Δ z H histogram. If no distinct peak is observed in the Δ z H histogram, then the JFP is considered to be zero. Table 1 also summaries the various distances obtained from both MCBJ and STM-BJ measurements. As shown in Table 1 , the JFP approaches 100% for molecules p-p-p, p-m-p, m-p-m and m-m-m. For molecule o-p-o, the JFP decreased sharply to 21% (MCBJ)/27% (STM-BJ) because the N in the terminal ortho pyridyl is partially hidden from the electrode surfaces and therefore it is difficult to form a bridge between the two gold electrodes [40] . Our inability to measure the conductance of o-m-o is explained by its short N---N length and the expected low conductance, which falls below the direct tunnelling conductance ( Supplementary Note 3 and Supplementary Fig. 13 ). The most-probable end-of-plateau electrode separations z H * follow the trends p-p-p >m-p-m >o-p-o, and p-m-p≈m-m-m that correlate with the molecular N---N distance, demonstrating that the gold-anchor link is primarily controlled by the gold–nitrogen bonds. Therefore, it is clear that changes in the position of the N atom within the anchors affects both the plateau length and the JFP, as well as the conductance. Quantum interference in the terminal and central rings For the linear molecules of group 1, both p-p-p and o-p-o have the same conductance value (10 −4.5 G 0 ) from the STM-BJ technique. The conductance value of o-p-o from MCBJ with the Gaussian fitting is 10 −5.0 G 0 , which is lower than that obtained using the STM-BJ. We also note that the width of the conductance peak in the 1D histogram from MCBJ measurements is bigger than that from the STM-BJ. This is associated with the different stretching of the molecular junctions during their formation using the two techniques, as verified by the 2D conductance properties (see Supplementary Information ). Nevertheless, compared with the STM-BJ results, the peak value from Gaussian fitting to MCBJ measurements is lower. These results suggest that a wider variety of configurations were formed between the molecule and electrodes during junction stretching in MCBJ measurements because of the higher stability, while some of the molecular configurations, especially the fully stretched configurations, could be monitored using the STM-BJ. The conductance of the m-p-m molecule was found to be lower than the other two group-1 members, with o-p-o and p-p-p in both the STM-BJ and MCBJ experiments, having a measured value of 10 −5.5 G 0 . Comparisons between the conductances of molecules in group 2 also demonstrate that the para/meta/ortho variations in the terminal ring result in only small conductance changes of less than an order of magnitude. The measured conductance of m-m-m is 10 −6.9 G 0 , which is lower than the p-m-p conductance of 10 −6.0 G 0 . However, as mentioned above, we were unable to measure any electrical properties of o-m-o from either MCBJ or STM-BJ owing to the masking direct tunnelling current. For comparison, in ref. 41 , changing from para to meta in the central ring of an OPV3 caused the conductance to drop by one order of magnitude, while in ref. 32 changing the position of an -SMe or an -NH 2 in the anchor groups from para to meta caused a change of almost two orders of magnitude. These are different anchor groups from ours, but the conductance changes are comparable with our experimental observations. To elucidate the measured conductance trends, we performed a density functional theory (DFT)-based optimization of each molecule using SIESTA [42] , [43] and carried out electron transport calculations using the approach discussed in our previous papers [30] , [39] . Unlike the p-p-p molecule, the other molecules possess anchoring nitrogen atoms located at meta or ortho positions within the terminal rings that do not naturally bind to planar electrode surfaces. To study the transport properties of these molecules, we attached the anchor nitrogen atoms to the apexes of pyramidal gold electrodes, as shown in Figs 3 and 4 and in Supplementary Note 5 , and Supplementary Fig. 14 . The molecules shown in these figures have been geometrically relaxed using SIESTA and it is clear that many of these geometries, such as the ma-m-ma conformation in Fig. 3 , would not tend to form a bridge between two opposing pyramids. We also note that molecular lengths ( L ), defined as the distance between the centres of the furthest non-hydrogen atoms in the molecule, are the same for these different conformations, whereas the N---N distance, which is the distance between the centres of the N atoms, does vary. Therefore, in Table 1 the largest N---N distance ( L NN ) of each molecule is calculated and compared with the most-probable electrode separation at the end of the high-conductance plateau, that is, z H *. 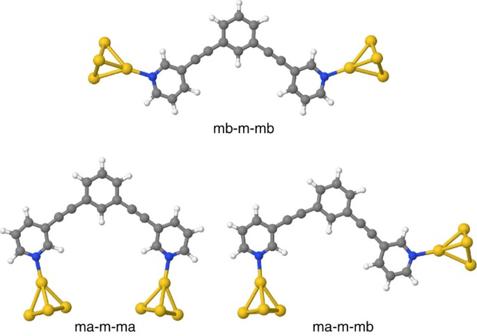Figure 3: Molecular conformations. Idealized junction geometries for the planar m-m-m molecule are shown. The N---N distance varies with conformations, therefore, the molecular N---N distance,LNNis defined as the largest N---N distance (mb-m-mb junction geometry). Figure 3: Molecular conformations. Idealized junction geometries for the planar m-m-m molecule are shown. The N---N distance varies with conformations, therefore, the molecular N---N distance, L NN is defined as the largest N---N distance (mb-m-mb junction geometry). 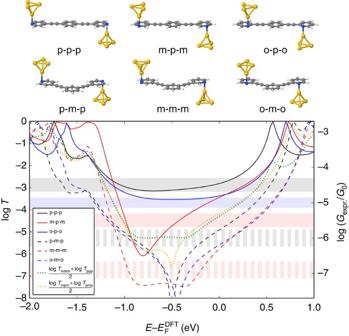Figure 4: Systematic junction geometries and transmission coefficient functions. The top figures show idealized junction geometries for all six molecules with the gold tip attached perpendicular to the pyridine ring. The bottom graphs show corresponding transmission coefficient curves. For comparison, the coloured and patterned horizontal shaded bars show the experimentally measured MCBJ values of log (G/G0) (right-hand scale). The thickness of the bars corresponds to the error bar of the experimental log (G/G0). These show that both the transmission coefficients around theEFand the experimental conductance values are separable into two groups corresponding to X-p-X and X-m-X connectivities. The green (yellow) dotted line is the average of logTmmmand logTppp(logTmpmand logTpmp). It should be noted that over most of the energy range from −0.8 to −0.4 eV, the m-m-m results have the lowest transmission coefficient. At these low transmissions, the contribution from the σ channel becomes comparable with that of the π channel and therefore in this energy range, the circuit rule is violated. Full size image Figure 4: Systematic junction geometries and transmission coefficient functions. The top figures show idealized junction geometries for all six molecules with the gold tip attached perpendicular to the pyridine ring. The bottom graphs show corresponding transmission coefficient curves. For comparison, the coloured and patterned horizontal shaded bars show the experimentally measured MCBJ values of log ( G/G 0 ) (right-hand scale). The thickness of the bars corresponds to the error bar of the experimental log ( G/G 0 ). These show that both the transmission coefficients around the E F and the experimental conductance values are separable into two groups corresponding to X-p-X and X-m-X connectivities. The green (yellow) dotted line is the average of log T mmm and log T ppp (log T mpm and log T pmp ). It should be noted that over most of the energy range from −0.8 to −0.4 eV, the m-m-m results have the lowest transmission coefficient. At these low transmissions, the contribution from the σ channel becomes comparable with that of the π channel and therefore in this energy range, the circuit rule is violated. Full size image The central focus of this section is to understand the relative contribution to the conductance from QI in the terminal and central aromatic rings, and to demonstrate that the quantum circuit rule is satisfied at the level of DFT. The largest value of z H * among all the measured molecules ( Table 1 ) was found to be z H *=1.80 nm for the p-p-p. The value of z H * for other molecules was typically shorter than this value. Therefore, the typical conductances occur when the molecules are not fully stretched and there is a possibility of metal-ring overlap between the gold electrode and the pyridyl rings. To analyse such events, we systematically constructed junction geometries with two 35-atom gold (111)-directed pyramids attached to the N atoms perpendicular to the pyridyl rings, as shown in Fig. 4 , and then computed the transmission coefficient curves T(E) for these geometries. (Alternative junction geometries are investigated in Supplementary Note 6 and Supplementary Figs 15–17 . Supplementary Figure 18 shows a comparison between theoretical and experimental conductances.) Figure 4 demonstrates that for a wide range of Fermi energy choice, the theoretical and experimental conductances of the X-p-X molecules of group 1 are distinctly higher than those of the molecules in group 2, as expected from previous studies [27] , [28] , [32] , [41] . Figure 4 also shows that for wide range of energies in the gap between the highest occupied molecular orbital (HOMO) and lowest unoccupied molecular orbital (LUMO), the ordering of the transmission coefficients follows the experimental conductance ordering. To demonstrate the resilience of the circuit rule, dotted lines are plots of (log T mmm +log T ppp )/2 and (log T mpm +log T pmp )/2. The similarity of these two curves shows that the product rule is satisfied over a wide range of energies within the HOMO-LUMO gap. To demonstrate that QI effects associated with variations in the positions of the N atoms are suppressed owing to the presence of a parallel conductance path associated with the electrode-ring overlap, we performed transport calculations in which we artificially set to zero every Hamiltonian and overlap matrix element that couples carbon and hydrogen atoms to gold atoms, leaving couplings between the nitrogen atoms and gold as the only possible transport path. The resulting transmission coefficients are shown as dashed lines in Fig. 5 and demonstrate that without metal-ring interactions the meta link in the terminal ring of the m-p-m molecule reduces the conductance by orders of magnitude, which is comparable with the effect of a meta link in the central ring, whereas in the presence of metal-ring interactions meta coupling in the terminal rings has a much smaller effect. 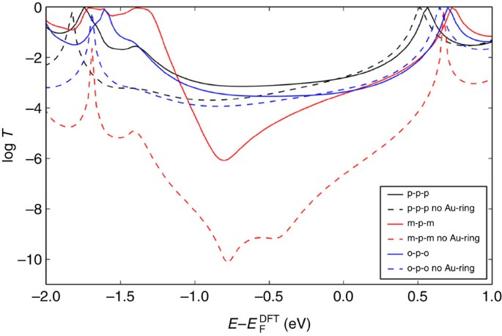Figure 5: Transmission curves with and without metal-ring coupling. The corresponding junction geometries are shown inFig. 4. Dashed lines are without metal-ring coupling, the continuous curves are with metal-ring coupling. Figure 5: Transmission curves with and without metal-ring coupling. The corresponding junction geometries are shown in Fig. 4 . Dashed lines are without metal-ring coupling, the continuous curves are with metal-ring coupling. Full size image Derivation of the quantum circuit rule for molecular conductances Having demonstrated that the effect of QI in a given ring depends on the position of the ring within the molecule (that is, whether it is a terminal or a central ring), we now derive the following quantum circuit rule describing the conductances of different ring combinations: This captures the property that the contribution to the conductance from the ring Y in molecules of type p-Y-p and m-Y-m are identical. To derive the circuit rule, consider the simple tight-binding model of Fig. 6b , in which three rings (labelled A, B and C) are coupled by nearest neighbour couplings α and β. To calculate the transmission coefficient arising when 1D electrodes are connected to site i of ring A and q of ring C, we first calculate the Green’s function G qi of the whole structure in the absence of the electrodes. 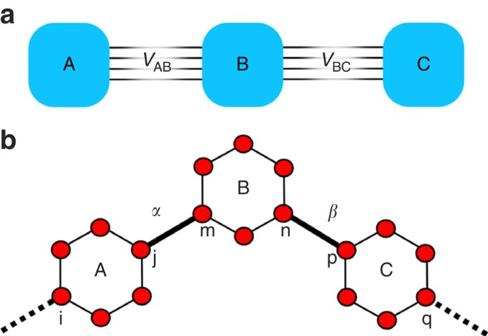Figure 6: Abstract models. (a) An abstract depiction of three coupled quantum subsystems. (b) A simple tight-binding model of the three ring system. (In the figure p-m-p connection is shown to illustrate the connecting sites i, j, m, n, p and q.) Figure 6: Abstract models. ( a ) An abstract depiction of three coupled quantum subsystems. ( b ) A simple tight-binding model of the three ring system. (In the figure p-m-p connection is shown to illustrate the connecting sites i, j, m, n, p and q.) Full size image This structure is an example of three arbitrary-coupled quantum objects shown schematically in Fig. 6a , whose Green’s function is given by Electron propagation from subsystem A to subsystem C is described by the block G CA , for which the above equation yields where g X =( E−H X ) −1 ( X =A or C) and . As an example, for the tight-binding model of Fig. 6b , this becomes G qi =( g C ) qp B nm ( g A ) ji , where and σ = α 2 ( g A ) jj ( g B ) mm + β 2 ( g C ) pp ( g B ) nn + α 2 β 2 ( g A ) jj ( g C ) pp [( g B ) nm ( g B ) mn −( g B ) nn ( g B ) mm ]. The crucial point is that B nm does not depend on the choice of p, q, i and j, because due to rotational symmetry, ( g A ) jj and ( g C ) pp are independent of j and p for any choice of j and p. This means that B nm does not depend on the choice of meta, ortho or para coupling for rings A and C and only depends on the connectivity of ring B. When the rings A and C are coupled to the electrodes, this rotational symmetry is broken slightly. However, provided E F lies in the HOMO-LUMO gap of A and C and the coupling to the electrodes is small (as is usually the case for molecules attached to gold electrodes, where the level broadening is much less than the level spacing), then the symmetry breaking is weak [26] . Since the electrical conductance is proportional to | G qi | 2 , this means that the electrical conductance G XYZ /G 0 of molecules of the type X-Y-Z is proportional to a product of the form a X × b Y × a Z and hence the quantum circuit rule is satisfied. The factors a X , b Y , a Z are contributions to the overall conductance from the separate rings, but it should be noted that they are not themselves individually measureable conductances. The above analysis can be easily applied to a molecule with two rings yield the circuit rule , where the G pp and G mm are the conductances of the molecule with para-para and meta-meta connected rings, and G pm is the conductance of the molecule with meta and para rings (see Supplementary Information for a DFT confirmation of this rule). To check the experimental validity of the circuit rule (1) for the OPEs of Fig. 1 , we examine the measured conductance values presented in Table 1 . For example, rearranging equation (1) into the form and substituting into the right-hand side, the measured values for G ppp , G mmm and G mpm yields G pmp =10 −5.9 G 0 , which compares well with the measured value of G pmp =10 −5.8 G 0 shown in Table 1 . We have presented charge transport studies of pyridyl terminated OPE derivatives, using the MCBJ and STM-BJ techniques, DFT-based theory and analytic Green’s functions, and have investigated the interplay between QI effects associated with central and terminal rings in molecules of the type X-Y-X. Our results demonstrated that the contribution to the conductance from the central ring is independent of the para or meta nature of the anchor groups and the combined conductances satisfy the quantum circuit rule G ppp / G pmp = G mpm / G mmm . For the simpler case of a two-ring molecule, the circuit rule is satisfied ( Supplementary Note 8 , and Supplementary Figs 19 and 20 ). It should be noted that the circuit rule does not imply that the conductance G XYX is a product of three measureable conductances associated with rings X, Y and X. Indeed the latter property does not hold for a single molecule. On the other hand, provided sample to sample fluctuations lead to a broad distribution of phases within an ensemble of measurements, a product rule for ensemble averages of conductances can arise. This possibility is discussed in detail in Supplementary Notes 7 and 9 . The qualitative relationship between the conductances agrees well with the simple QI picture of molecular conduction. It has been reported that destructive QI exists in benzene with the meta connectivity and is responsible for the observed reduction of conductance [16] , [20] , [28] , whereas for para and ortho connectivities, constructive QI should be observed [44] , [45] . The transmission coefficient calculations through junctions where the metal-ring connection is artificially blocked ( Fig. 5 ) show that the artificially coupled pyridyl ring exhibits similar behaviour to the benzene ring, with destructive QI in the case of the meta coupling significantly reducing the conductance compared with para and ortho connectivities. The dashed curves in the bottom panel in Fig. 5 clearly demonstrate that when the conduction is through only the nitrogen atoms, the conductance of the meta isomer is much lower than in the para and ortho isomers. More realistically, however, in the presence of metal-ring overlap, the effect of varying the positions of the nitrogens in the anchors becomes much weaker, and as demonstrated by Fig. 4 the major changes in the molecular conductance are caused by the variations in the connectivity of the central ring. The dominant influence of the central ring is accounted for by the fact that the central ring is not in direct contact with electrodes and therefore no parallel conductance paths are present, which could bypass the ethynylene connections to the anchors. In a subnanometre scale molecular circuit, as in standard complementary metal-oxide-semiconductor (CMOS) circuitry, electrical insulation is of crucial importance. Destructive interference in a two-terminal device may not be desirable, because of the lower conductance. However, for a three-terminal device minimizing the conductance of the third terminal is highly desirable, because the third (gate) electrode should be placed as close to the molecule as possible, but at the same time, there should be no leakage current between the molecule and gate. One way of achieving this may be to use an anchor group with built-in destructive interference. Therefore, destructive QI may be a vital ingredient in the design of future three-terminal molecular devices and more complicated networks of interference-controlled molecular units. Conductance measurements The transport characteristics in single-molecule junctions were studied by MCBJ and STM-BJ measurements in solution at room temperature. The latter contained typically 0.1 mM of the OPE-type molecules in a mixture of 1,3,5-trimethylbenzene (Aldrich, p.a.) and tetrahydrofuran (Aldrich, p.a), 4:1 (v/v). MCBJ measurements The MCBJ experiments are based on the formation and breaking of a nanogap between a notched, freely suspended gold wire (0.1 mm diameter, 99.999%, Goodfellow), fixed on spring steel sheets (10 mm × 30 mm, thickness 0.25 mm) with a two-component epoxy glue (Stycast 2850 FT with catalyst 9). The sample sheets were fixed between two holders. A Kel-F liquid cell with a Kalrez O-ring was mounted onto the sheet. During the measurements, the steel sheet could be bent with a pushing rod, which was controlled by a combination of a stepper motor and a piezo stack. The bending was initialized by the stepper motor. Once the measured current decreased to a value corresponding to 15 G 0 , the stepper motor stops moving and the piezo stack was activated. This strategy reduced significantly noise contributions from the operation of the stepper motor. The movement of the piezo stack controlled the breaking and the reformation of nanoscale contacts, typically in the range between the noise threshold ( G <10 −8 G 0 ) and a high-conductance limit, which was set to 10 G 0 . Molecular junctions could form upon breaking the gold–gold nanocontacts. The entire cycle was repeated for >1,000 times to obtain statistically relevant data. In the MCBJ setup, the current could be recorded as a feedback signal at a given bias voltage (typically between 0.020 and 0.200 V). The two ends of the ‘broken wire’ were taken as working electrodes WE1 and WE2. The MCBJ unit is controlled by a lab-built bipotentiostat with two bipolar tunable logarithmic I – V converters as current measuring units, which are operated by a custom-designed microcontroller. The system provides the following three analogue signals: the potential of WE1, the voltage difference between the two working electrodes WE1 and WE2 (bias voltage V bias ), driving the current through the two gold electrodes for the conductance measurements, and the voltage output of the piezo stack in the range of 0–50 V, allowing the displacement of the piezo stack up to 8 μm with rates ranging from 3 to 3,000 nm s −1 . The latter translates into lateral pulling (pushing) rates between the two gold leads of 0.1–100 nm s −1 . The distance between the two gold electrodes in the MCBJ setup was calibrated with complementary STM-BJ experiments, assuming that the tunnelling decay is identical under the same experimental conditions. Further technical details of the MCBJ setup was reported by Hong et al . [46] STM-BJ The STM-BJ technique repeatedly traps molecules between a sharp STM tip and an atomically flat sample. The STM-BJ measurements were carried out with a molecular imaging PicoSPM housed in an all-glass argon-filled chamber and equipped with a dual preamplifier capable of recording currents in a wide range of 1 pA to 150 μA with high resolution. The non-amplified low-current signal was fed back to the STM controller preserving the STM imaging capability. The current–distance measurements were performed with a separate, lab-built analogue ramp unit. For further technical details, we refer to our previous work [47] , [48] . The sample electrode was gold single-crystal bead. The Au (111) facet before each experiment was subjected to electrochemical polishing and annealing in a hydrogen flame followed by cooling under Ar. A freshly prepared solution containing typically 0.1 mM of the respective molecule was added to a Kel-F flow-through liquid cell mounted on top of the sample, and the uncoated STM tip was electrochemically etched using gold wire (Goodfellow, 99.999%, 0.25 mm diameter) capable of imaging with atomic resolution. This system relies on trapping a molecule between the end of an Au tip and the gold substrate. After assembling the experiment, the following protocols were applied: the tip was brought to a preset tunnelling position typically defined by i T =50–100 pA and a bias voltage V bias of 0.10, 0.065 and 0.175 V, followed by imaging the substrate. After fixing the lateral position of the tip, the STM feedback is switched off and current–distance measurements were performed, and then the vertical movement of the tip was controlled by the ramp unit. The measuring cycle was performed in the following way: the controlling software drives the tip towards the adsorbate-modified surface. The approach was stopped when a predefined upper current limit was reached (typically 10 μA or <10 G 0 with G 0 being the fundamental conductance quantum 77.5 μS). After a short delay (~100 ms) ensuring tip relaxation and the formation of stable contacts, the tip was retracted by 2–5 nm until a low current limit of ~10 pA was reached. The approaching and withdrawing rates were varied from 56 to 145 nm s −1 . The entire current–distance traces were recorded with a digital oscilloscope (Yokogawa DL 750, 16 bit, 1 MHz sampling frequency) in blocks of 186 individual traces. Up to 2,000 traces were recorded for each set of experimental conditions to guarantee the statistical significance of the results. For each molecule, the data were acquired at three different bias voltages of 0.065, 0.100 and 0.175 V. Theory and simulations All molecules in this study were first geometrically optimized in isolation. For molecules with meta and ortho terminal pyridyl rings, all the non-equivalent planar conformations were geometrically relaxed. All geometrical optimizations were carried out using the DFT code SIESTA, with a generalized gradient approximation method (PBE functional), double-zeta polarized basis set, 0.01 eV Å −1 force tolerance and 250 Ry mesh cutoff. To investigate ideal junction geometries, a small four-atom gold pyramid was attached to the N atoms of the molecules, with Au–N–C angle being 120° and Au–N bond length being 2.1 Å, as shown in Supplementary Fig. 14 . Many of these junction geometries are unlikely to happen in BJ experiments, and during the junction elongation typically the gap between the electrodes is shorter than the molecular length. We constructed another set of idealized junction geometries where the gold pyramid is attached to rings from the side, perpendicular to the ring. These junction geometries are shown in Fig. 4 . For transport calculation, the four-atom gold pyramids that are seen in Fig. 4 are extended to a 35-atom gold pyramid. Transmission coefficients were computed using the GOLLUM code [49] . In break-junction experiments, more complicated structures are expected. For this reason, we also carried out BJ simulations using the approach discussed in our previous papers [30] , [39] . The geometrically optimized molecules were inserted between two opposing 35-atom (111) directed pyramids with four different tip separations. (The tip separation is defined to be the centre to centre distance between the apex atoms of the two opposing pyramids.) In the initial geometries, the molecules were shifted slightly towards one of the pyramids and the initial Au–N distances were ~2.5 Å. Then the constructed structure was geometrically relaxed such that the base layers of the pyramids were kept fixed during the optimizations. Optimized junction geometries are shown in Supplementary Figs 16 and 17 . To produce the conductance-trace curves in Supplementary Fig. 18 , the transmission coefficient T(E) was calculated for each relaxed junction geometry, by first obtaining the corresponding Hamiltonian and then overlapping matrices with SIESTA and double-zeta polarized basis set. The transmission coefficient for all junction geometries in this study was calculated using wide-band electrodes with Γ=4.0 eV. The wide-band electrodes were coupled to the two base layers of gold atoms of the 35-atom pyramids. A few additional transmission coefficient functions can be seen in Supplementary Fig. 15 . To produce conductance-trace curves, the transmission coefficient T(E) was calculated for each relaxed junction geometry and the conductance G/G 0 = T(E F ) was obtained by evaluating T(E) at the Fermi energy E F . A value of E F =−0.65 eV, relative to the bare DFT Fermi energy ( E F DFT ) was chosen to account for the expected LUMO level shift, as discussed in ref. 39 , where the Fermi energy shift was adjusted to match measured and computed conductance for the pyridine-terminated oligoyne molecules. Synthesis Details of the synthesis are in the Supplementary Note 1 . How to cite this article: Manrique, D. Z. et al . A quantum circuit rule for interference effects in single-molecule electrical junctions. Nat. Commun . 6:6389 doi: 10.1038/ncomms7389 (2015).